Endogenous fructose production and metabolism in the liver contributes to the development of metabolic syndrome Carbohydrates with high glycaemic index are proposed to promote the development of obesity, insulin resistance and fatty liver, but the mechanism by which this occurs remains unknown. High serum glucose concentrations are known to induce the polyol pathway and increase fructose generation in the liver. Here we show that this hepatic, endogenously produced fructose causes systemic metabolic changes. We demonstrate that mice unable to metabolize fructose are protected from an increase in energy intake and body weight, visceral obesity, fatty liver, elevated insulin levels and hyperleptinaemia after exposure to 10% glucose for 14 weeks. In normal mice, glucose consumption is accompanied by aldose reductase and polyol pathway activation in steatotic areas. In this regard, we show that aldose reductase-deficient mice are protected against glucose-induced fatty liver. We conclude that endogenous fructose generation and metabolism in the liver represents an important mechanism by which glucose promotes the development of metabolic syndrome. There is increasing evidence that excessive intake of carbohydrates may have a role in the epidemic of obesity and insulin resistance. Low-carbohydrate diets have been found effective at inducing weight loss, often with improvement in hypertriglyceridaemia and insulin resistance [1] , [2] , [3] , [4] , [5] . One of the postulated mechanisms revolves around the fructose content of carbohydrate-containing foods [6] , [7] , [8] . Fructose, present in added sugars, such as sucrose and high-fructose corn syrup, can induce all of the features of metabolic syndrome in animals, and the metabolic effects occur independently of excessive energy intake [9] . In previous studies, when rats are pair-fed either fructose or glucose as part of their diet, the fructose-fed rats show worse features of metabolic syndrome [10] , [11] . Similarly, in humans the administration of beverages containing 25% fructose to overweight individuals also causes more visceral obesity and insulin resistance compared with subjects administered 25% glucose [12] . Studies such as these suggest it is the fructose content in added sugars, which may account for why sugary soft drinks are so strongly linked with the development of obesity, fatty liver and insulin resistance [13] , [14] , [15] , [16] , [17] , [18] . At present, there is a vast literature suggesting that carbohydrates with a high glycaemic index increase the risk for obesity and insulin resistance [19] , [20] . The glycaemic index relates to the ability of carbohydrates to increase plasma glucose levels following ingestion, for which glucose carries the highest level (1.0), whereas fructose has a low glycaemic index (0.2) [21] . Whether high glycaemic index carbohydrates increase the risk for insulin resistance beyond that associated with increased energy intake has been controversial [2] , [22] . However, a recent study reported that a diet low in high glycaemic carbohydrates may help maintain weight loss independently of energy intake [23] . Many high glycaemic foods also contain fructose. For instance, sucrose is a disaccharide of glucose and fructose, and high-fructose corn syrup is a mixture of glucose and fructose, raising the question of whether fructose is responsible for the effects of high glycaemic foods to increase the risk for metabolic syndrome [24] . To further complicate this issue, fructose can be generated endogenously via the polyol pathway from glucose. Specifically, aldose reductase (AR) metabolizes glucose to sorbitol, which can then be converted to fructose by sorbitol dehydrogenase. Thus, if AR were highly expressed or activated in the liver, some of the glucose absorbed might be converted to fructose, and hence possibly provide a mechanism for inducing features of the metabolic syndrome. To test this hypothesis, we provided drinking water with or without glucose (10% (wt/vol)) to wild–type (WT) mice or fructokinase (ketohexokinase, KHK) knockout (KO) mice for 14 weeks. We selected 14 weeks based on our previous studies on mice drinking fructose [25] . Parallel groups of mice were also maintained on regular chow (containing 60% carbohydrate and no fructose). We have previously shown that fructokinase KO mice (KHK-A/C KO) have a normal phenotype [26] and are protected from fructose-induced metabolic syndrome [25] . Importantly, fructokinase does not metabolize glucose [27] . In this study we show that there is a significant activation of AR and the polyol pathway in the liver of mice exposed to drinking glucose (10% in water), which leads to the production of ‘endogenous fructose’, and that the blockade of its metabolism in fructokinase-deficient mice exerts protection against glucose-induced fatty liver and insulin resistance. Similar glucose intake in WT and KHK-A/C-deficient mice As shown in Fig. 1 , both WT and KHK-A/C KO mice ingested similar amounts of glucose water (cumulative, Fig. 1a ). Both glucose-fed groups reduced their chow intake in response to the energy intake from glucose ( Fig. 1b , left). However, the reduction in chow intake was not enough to compensate for the energy intake from the glucose water and, hence, both groups remained in positive energy balance ( Fig. 1b , left). Nevertheless, the KHK-A/C KO mice reduced their chow intake more and, hence, their total energy intake was lower than that observed in WT mice fed glucose ( Fig. 1b , left). Measurements of urinary fructose and glucose are also included ( Supplementary Fig. S1A, B ), as KHK-A/C KO mice are known to excrete increased levels of urinary fructose. However, the amount of energy loss via the urine was minor and did not alter the energy balance results. 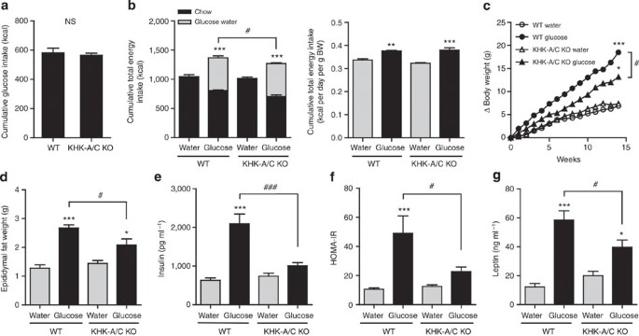Figure 1: Effect of glucose consumption on metabolic parameters in WT and KHK-A/C KO mice. WT mice and KHK-A/C KO mice were provided drinking water containing 10% glucose or tap water with normal mouse chowad libitumfor 14 weeks (n=6 per group). (a) Cumulative energy intake of glucose water for 14 weeks. (b) Left: cumulative total energy intake of chow diet with 10% glucose water or tap water for 14 weeks. Right: total energy intake per gram body weight (BW) per day of normal chow diet with 10% glucose water or tap water for 14 weeks. (c) Growth curves of WT mice and KHK-A/C KO mice. Epididymal fat weight (d). Serum insulin (e). HOMA-IR (f). Serum leptin (g). Data represent means±s.e.m. *P<0.05, **P<0.01, ***P<0.001 versus respective water control.#P<0.05.###P<0.001 (analysis of variance, Tukey’spost hoctest). Figure 1: Effect of glucose consumption on metabolic parameters in WT and KHK-A/C KO mice. WT mice and KHK-A/C KO mice were provided drinking water containing 10% glucose or tap water with normal mouse chow ad libitum for 14 weeks ( n =6 per group). ( a ) Cumulative energy intake of glucose water for 14 weeks. ( b ) Left: cumulative total energy intake of chow diet with 10% glucose water or tap water for 14 weeks. Right: total energy intake per gram body weight (BW) per day of normal chow diet with 10% glucose water or tap water for 14 weeks. ( c ) Growth curves of WT mice and KHK-A/C KO mice. Epididymal fat weight ( d ). Serum insulin ( e ). HOMA-IR ( f ). Serum leptin ( g ). Data represent means±s.e.m. * P <0.05, ** P <0.01, *** P <0.001 versus respective water control. # P <0.05. ### P <0.001 (analysis of variance, Tukey’s post hoc test). Full size image As animals gain weight their energy requirements increase, thus requiring a re-evaluation of energy intake factored for weight. In this regard, both WT and KHK-A/C KO mice receiving glucose had greater total energy intake than mice drinking only water, but there was no difference between the glucose-fed WT and KHK-A/C KO mice based on calculations of daily intake, as well as cumulative energy intake ( Fig. 1b , right). KHK deficiency blocks metabolic syndrome in mice WT mice drinking glucose water showed significant weight gain, visceral (epididymal) fat accumulation, hyperinsulinaemia and elevated HOMA-IR (homeostasis model assessment insulin resistance), and hyperleptinaemia compared with WT mice receiving water ( Fig. 1c–g ). KHK-A/C KO mice given glucose also gained weight, visceral fat and developed elevated leptin levels compared with KHK-A/C KO mice on regular water, although levels of insulin and HOMA-IR were not different ( Fig. 1c–g ). Nevertheless, KHK-A/C KO mice receiving glucose had significantly less weight gain, visceral obesity, hyperinsulinaemia, HOMA-IR and hyperleptinaemia compared with glucose-fed WT mice ( Fig. 1c–g ). Of interest, despite having different insulin levels, no differences were observed between WT and KHK-A/C KO mice receiving glucose in insulin tolerance and hepatic glucokinase expression ( Supplementary Figs S2 and S3 ). WT and KHK-A/C KO mice receiving glucose showed higher glycated haemoglobin A1C, higher total and low-density lipoprotein cholesterol and lower blood urea nitrogen (BUN) levels compared with control mice receiving regular drinking water ( Supplementary Table S1 ). However, there were no differences in these parameters between the glucose-fed WT and KHK-A/C KO mice. Serum creatinine, triglycerides and high-density lipoprotein cholesterol did not differ among the four groups of mice. KHK deficiency blocks glucose-induced fatty liver in mice WT mice receiving glucose developed enlarged livers that were grossly pale; these changes were not observed in the glucose-fed KHK-A/C KO mouse ( Fig. 2a,b ). Histologically, haematoxylin and eosin (H&E)-stained sections and Oil red O staining documented the presence of steatosis ( Fig. 2c,d and Supplementary Table S2 ). H&E staining of the livers of WT mice fed glucose water showed that macrovesicular steatosis was dominant around the portal triad (zone 1) and into the adjoining midzonal area (zone 2), whereas microvesicular lipid accumulation occurred near the central vein (zone 3) and also extended into the adjoining midzonal area ( Fig. 2d and Supplementary Table S2 ). In contrast, KHK-A/C KO animals on the high-glucose diet showed neither macro- nor microsteatosis, and similarly neither types of steatosis were observed in the control WT or KHK-A/C KO mice on tap water. The increased lipid deposition in glucose-fed WT mice was shown to be due to increased intrahepatic triglyceride, but not cholesterol, content ( Fig. 2e,f ). 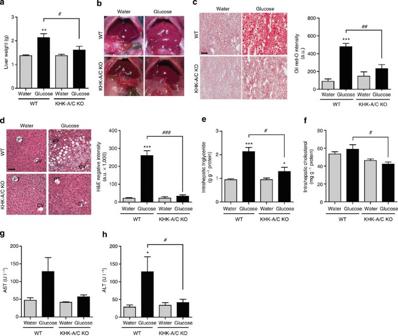Figure 2: Effect of glucose consumption on liver histology and function. WT mice and KHK-A/C KO mice were given 10% glucose water, or tap water for 14 weeks with normal chow dietad libitum(n=6 per group). (a) Liver weight. (b) Gross images of liver showing increased liver size and pale colour in WT but not in KHK-A/C KO mice given glucose (size bar: 1 cm). (c) Representative images of oil red O staining, demonstrating increased fat accumulation (red) in WT but not in KHK-A/C KO mice given glucose (size bar 50 μM). (d) Representative images of H&E staining showing areas of macrosteatosis (white vesicles) in zone 2 and microsteatosis in zone 1 (surrounding the central vein, CV) in WT but not in KHK-A/C KO mice given glucose. PT, portal triad. (e) Intrahepatic triglyceride levels (size bar 50 μM). (f) Intrahepatic cholesterol levels. (g) Serum AST levels. (h) Serum ALT levels. Data represent means±s.e.m. *P<0.05, **P<0.01, ***P<0.001 versus respective water control.#P<0.05.##P<0.01.###P<0.001 (analysis of variance, Tukey’spost hoctest). Figure 2: Effect of glucose consumption on liver histology and function. WT mice and KHK-A/C KO mice were given 10% glucose water, or tap water for 14 weeks with normal chow diet ad libitum ( n =6 per group). ( a ) Liver weight. ( b ) Gross images of liver showing increased liver size and pale colour in WT but not in KHK-A/C KO mice given glucose (size bar: 1 cm). ( c ) Representative images of oil red O staining, demonstrating increased fat accumulation (red) in WT but not in KHK-A/C KO mice given glucose (size bar 50 μM). ( d ) Representative images of H&E staining showing areas of macrosteatosis (white vesicles) in zone 2 and microsteatosis in zone 1 (surrounding the central vein, CV) in WT but not in KHK-A/C KO mice given glucose. PT, portal triad. ( e ) Intrahepatic triglyceride levels (size bar 50 μM). ( f ) Intrahepatic cholesterol levels. ( g ) Serum AST levels. ( h ) Serum ALT levels. Data represent means±s.e.m. * P <0.05, ** P <0.01, *** P <0.001 versus respective water control. # P <0.05. ## P <0.01. ### P <0.001 (analysis of variance, Tukey’s post hoc test). Full size image Trichrome stain analysis demonstrated a small amount of collagen deposition in the periportal sinusoids of the high-glucose-fed WT animals ( Supplementary Fig. S4 ) without evidence for inflammation or other pathological alterations ( Supplementary Table S2 ). Mild elevation in transaminase levels was also present in the glucose-fed WT mice, as noted by elevated serum aspartate aminotransferase (AST) and serum alanine aminotransferase (ALT) levels ( Fig. 2g,h ). Western blotting of the liver tissue documented an increased expression of enzymes involved in fat synthesis (ATP citrate lyase (ACL) and fatty acid synthase (FAS)) in the glucose-fed WT mice compared with control WT mice ( Fig. 3a,b and Supplementary Fig. S5 ). Glucose-fed KHK-A/C KO mice showed a lower level of ACL compared with glucose-fed control mice. In addition, glucose-fed KHK-A/C KO mice had a tendency for lower FAS levels compared with glucose-fed WT mice, and also more evidence for active fatty acid oxidation, as noted by higher intrahepatic β-hydroxybutyrate levels ( Fig. 3c ). Of interest, changes observed at the protein levels of these lipogenic genes correlated with changes of these genes at the mRNA level ( Supplementary Fig. S6 ). These studies document that glucose-induced fatty liver is almost entirely mediated by fructokinase. 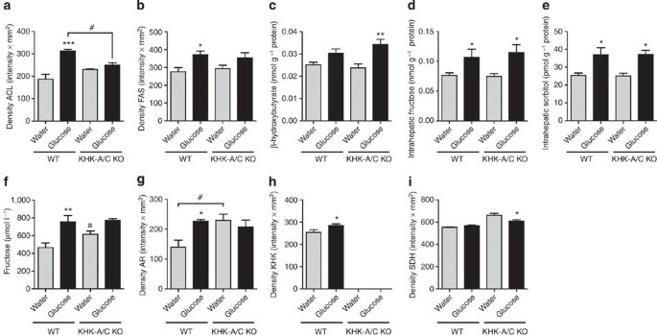Figure 3: Effect of glucose consumption on liver enzymes. (a,b) Western blot analysis of ACL (a) and FAS (b). Relative intensity to β-actin in liver (n=5), (full-length image of representative western blot analysis inSupplementary Fig. S5). (c) Serum β-hydroxy butyrate concentration (n=6). (d) Hepatic fructose content. (e) Hepatic sorbitol content. (f) Serum fructose concentration. (g–i) Western blot analysis of AR (g), KHK (h) and SDH (i). Relative intensity to β-actin in the liver (n=5), (full-length image of representative western blot inSupplementary Fig. S5). Data represent means±s.e.m. *P<0.05, **P<0.01 versus respective water control (analysis of variance, Tukey’spost hoctest);a,P<0.05 versus WT water by Student’st-test,#P<0.05, ***P<0.001. Figure 3: Effect of glucose consumption on liver enzymes. ( a , b ) Western blot analysis of ACL ( a ) and FAS ( b ). Relative intensity to β-actin in liver ( n =5), (full-length image of representative western blot analysis in Supplementary Fig. S5 ). ( c ) Serum β-hydroxy butyrate concentration ( n =6). ( d ) Hepatic fructose content. ( e ) Hepatic sorbitol content. ( f ) Serum fructose concentration. ( g – i ) Western blot analysis of AR ( g ), KHK ( h ) and SDH ( i ). Relative intensity to β-actin in the liver ( n =5), (full-length image of representative western blot in Supplementary Fig. S5 ). Data represent means±s.e.m. * P <0.05, ** P <0.01 versus respective water control (analysis of variance, Tukey’s post hoc test); a , P <0.05 versus WT water by Student’s t -test, # P <0.05, *** P <0.001. Full size image Activation of the polyol pathway in glucose-fed mice The observation that KHK-A/C KO mice were protected from glucose-mediated metabolic effects suggests that some of the glucose was being converted to fructose in the liver by the polyol pathway. Consistent with this hypothesis, we found elevated levels of fructose and sorbitol in the liver of WT mice given glucose water compared with mice given regular water ( Fig. 3d,e ). Serum fructose levels were also higher in glucose-fed WT mice compared with WT controls ( Fig. 3f ). This increase in hepatic fructose and sorbitol levels was accompanied by a higher expression of AR and KHK expression in WT mice when analysed by western blotting; however, the sorbitol dehydrogenase (SDH) level was not increased ( Fig. 3g–i and Supplementary Fig. S5 ). Of interest, KHK-A/C KO mice showed a higher AR expression, perhaps as a compensatory mechanism to the lack of KHK. In addition, KHK-A/C KO mice fed glucose had higher hepatic fructose and sorbitol levels compared with that of KHK-A/C KO mice on tap water. To determine whether the injured areas corresponded with the sites of expression of the polyol pathway, we performed immunofluorescence studies employing specific antibodies. As shown in Supplementary Figs S7 and S8 , both AR and KHK are predominantly expressed in zones 2 and 3 in glucose-fed animals correlating with the areas of severe hepatic steatosis. However, we also observed AR and KHK upregulation in zone 1 surrounding the portal triad. To evaluate the importance of the polyol pathway in the mechanism by which glucose induces hepatic steatosis, we gave 10% glucose to AR-deficient mice (ARKO) for 14 weeks and analysed intrahepatic levels of sorbitol and fructose. As shown in Fig. 4 , similar to our previous result in WT and KHK-A/C KO mice, ARKO mice drinking glucose had greater total energy intake compared with mice drinking tap water, which was not different compared with WT siblings drinking glucose ( Fig. 4a ). Of interest, ARKO mice drinking glucose had reduced body, liver and fat weight compared with that of WT mice ( Fig. 4b,c and Supplementary Figs S9 and S10 ). As expected, ARKO mice did not accumulate sorbitol ( Fig. 4d ) and fructose ( Fig. 4e ) intrahepatically compared with WT mice receiving water, indicating that the polyol pathway was responsible for the generation of endogenous fructose in mice drinking glucose. Consistent with reduced liver weight in ARKO mice drinking glucose, these mice had reduced fatty liver as denoted by a lower intrahepatic triglyceride concentration, H&E staining and Oil red O determination ( Fig. 4f and Supplementary Fig. S10 ). Moreover, serum of AST and ALT were not upregulated in the serum of ARKO mice drinking glucose compared with that of WT siblings ( Fig. 4g,h ). Furthermore, exposure of human HepG2 cells to high glucose levels (20 mM) resulted in a significant intracellular triglyceride accumulation that was prevented with an AR inhibitor, sorbinil (10 μM, Supplementary Fig. S11 ). Of interest, and as shown in the Supplementary Fig. S11 , the addition of fructose blocked the inhibitory effect of sorbinil on glucose-induced triglyceride accumulation in a dose-dependent manner. It is important to note that AR has already been implicated in the pathogenesis of fatty liver in diabetic animal models [28] , [29] , another condition in which the polyol pathway has been implicated. 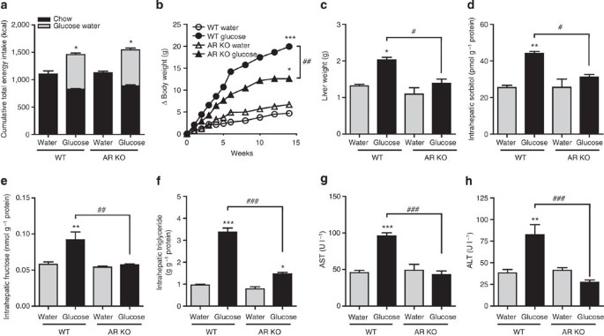Figure 4: ARKO mice do not develop glucose-induced fatty liver. WT mice and AR KO givenad libitumnormal chow diet with 10% glucose water, or tap water for 14 weeks (n=3–4). (a) Cumulative total energy intake of chow diet with 10% glucose water or tap water for 14 weeks. (b) Growth curves of WT mice and AR KO mice. (c) Liver weight. (d) Hepatic sorbitol content. (e) Hepatic fructose content. (f) Intrahepatic triglyceride levels. (g) Serum aspartate aminotransferase (AST) levels. (h) Serum alanine aminotransferase (ALT) levels. Data represent means±s.e.m. *P<0.05, **P<0.01, ***P<0.001 versus respective water control.#P<0.05.##P<0.01.###P<0.001 (analysis of variance, Tukey’spost hoctest). Figure 4: ARKO mice do not develop glucose-induced fatty liver. WT mice and AR KO given ad libitum normal chow diet with 10% glucose water, or tap water for 14 weeks ( n =3–4). ( a ) Cumulative total energy intake of chow diet with 10% glucose water or tap water for 14 weeks. ( b ) Growth curves of WT mice and AR KO mice. ( c ) Liver weight. ( d ) Hepatic sorbitol content. ( e ) Hepatic fructose content. ( f ) Intrahepatic triglyceride levels. ( g ) Serum aspartate aminotransferase (AST) levels. ( h ) Serum alanine aminotransferase (ALT) levels. Data represent means±s.e.m. * P <0.05, ** P <0.01, *** P <0.001 versus respective water control. # P <0.05. ## P <0.01. ### P <0.001 (analysis of variance, Tukey’s post hoc test). Full size image Role of energy intake in fructose-induced metabolic effects These studies show that glucose-mediated obesity, visceral fat accumulation, hyperinsulinaemia, hyperleptinaemia and fatty liver are all dependent in part on the conversion of glucose to fructose in the liver with the metabolism of fructose by KHK. In other words, the mechanism by which glucose induces its metabolic effects is largely dependent on fructose metabolites resulting from the fructose generated from glucose by the polyol pathway. Some of the protection that occurred in glucose-fed KHK-A/C KO mice can be attributed to a better control of the overall energy intake, as KHK-A/C KO mice had a lower energy intake due to a greater reduction in chow intake in response to similar glucose intake. To address the relative role of energy intake in mediating the KHK-dependent effects, we performed a subset analysis by comparing glucose-fed WT mice and glucose-fed KHK-A/C KO mice that had nearly identical glucose and total energy intake ( n =4 per group, Fig. 5a,b ). In these mice, significant differences were still noted in the degree of fatty liver and serum insulin levels ( Fig. 5c–f ), whereas no difference was shown in overall weight, visceral fat accumulation or leptin levels ( Supplementary Table S3 ). These studies suggest that glucose causes fatty liver and insulin resistance almost completely because of the conversion of glucose to fructose and that the effect of fructose to cause these metabolic effects does not require excessive energy intake. These studies are consistent with our observation that we can induce fatty liver, insulin resistance and frank diabetes in rats with a sucrose (40%) diet even when caloric intake is reduced to 90% of normal intake [30] . 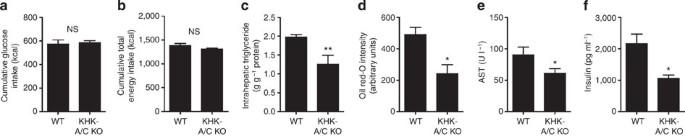Figure 5: Analysis of mice matched for glucose and total energy intake. WT mice and KHK-A/C KO mice were give 10% glucose water for 14 weeks with normal chow dietad libitum(n=4 per group). (a) Cumulative glucose intake (n=4). (b) Cumulative total energy intake (n=4). (c) Intrahepatic triglyceride levels (n=4). (d) Quantification of oil red O staining (n=4). (e) Serum aspartate aminotransferase (AST) levels (n=4). (f) Serum insulin levels (n=4). Data represent means±s.e.m. *P<0.05, **P<0.01 by Student’st-test. NS, not significant (analysis of variance, Tukey’spost hocanalysis). Figure 5: Analysis of mice matched for glucose and total energy intake. WT mice and KHK-A/C KO mice were give 10% glucose water for 14 weeks with normal chow diet ad libitum ( n =4 per group). ( a ) Cumulative glucose intake ( n =4). ( b ) Cumulative total energy intake ( n =4). ( c ) Intrahepatic triglyceride levels ( n =4). ( d ) Quantification of oil red O staining ( n =4). ( e ) Serum aspartate aminotransferase (AST) levels ( n =4). ( f ) Serum insulin levels ( n =4). Data represent means±s.e.m. * P <0.05, ** P <0.01 by Student’s t -test. NS, not significant (analysis of variance, Tukey’s post hoc analysis). Full size image These studies suggest that under certain conditions glucose may induce metabolic syndrome in mice via an AR, fructose-dependent pathway. Whether this is occurring in humans ingesting high glycaemic foods remains to be determined. However, as in mice, AR can be activated in humans by a number of ways, including by high glucose concentrations. Total parenteral nutrition, in which a 35% glucose solution is provided by the vein, is associated with the development of fatty liver, and experimental studies have shown that it is mediated by the glucose component of the infused fluids [31] , [32] . Soft drinks containing high-fructose corn syrup also deliver markedly high-glucose solutions (4–6%) to the gut, and sucrose-containing soft drinks provide similar amounts of glucose after the sucrose is degraded in the intestine. Thus, soft drinks are a special problem, as they provide both fructose and glucose together, in which the presence of glucose is also known to enhance fructose absorption [33] . It is thus not surprising that soft drink intake is associated with an increased risk for obesity, fatty liver and insulin resistance [13] , [14] , [15] , [16] , [17] , [18] , [34] , [35] . Furthermore, in a randomized study of overweight subjects, the administration of sugary soft drinks (1 litre per day) for 6 months was associated with significantly more visceral fat, hepatic fat and serum triglycerides compared with groups given diet soda, milk or water [36] . In conclusion, the mechanism by which glucose causes weight gain, fat accumulation, fatty liver and insulin resistance is largely due to activation of AR in the liver with conversion of glucose to fructose. Although some of these effects are due to the ability of fructose to increase energy intake, the effect of fructose to induce insulin resistance and fatty liver is independent of energy intake. These studies provide new insights into how carbohydrates may cause obesity, fatty liver and insulin resistance. Animal study KHK-A/C KO mice, which were of C57BL/6 background and were lacking both ketohexokinase-A and ketohexokinase-C, were generated as described previously [37] , [38] . KHK-A/C KO homozygous mice and WT littermates (male, 10-week-old) were used. They were maintained in a temperature- and humidity-controlled specific pathogen-free condition on a 14-h dark/10-h light cycle, and were allowed ad libitum access to normal laboratory chow (Harlan Teklad, 2920X). WT mice and KHK-A/C KO mice were assigned to the control group or the glucose water group ( n =6), matching the mean body weight among the groups. Mice had free access to normal laboratory chow and water containing 10% glucose or tap water for 14 weeks. Glucose water was prepared by dissolving D -(+)-glucose (Sigma-Aldrich) in tap water. Body weight was measured every week, and energy intake from both normal chow and glucose water was measured two times per week. Urine samples were collected at 12 weeks. Mice were killed after 6 h fasting of food and glucose water. Blood were withdrawn, and tissues were taken and frozen in liquid nitrogen. ARKO in the C57BL/E background were obtained from Jackson Laboratory (Bar Harbor, ME) and bred in our institution in a temperature- and humidity-controlled specific pathogen-free condition on a 14-h dark/10-h light cycle, and were allowed ad libitum access to normal laboratory chow (Harlan Teklad, 2920X). The experimental procedure was similar to the one explained above for KHK-A/C KO mice. All experiments were conducted with adherence to the NIH Guide for the Care and Use of Laboratory Animals. The animal protocol was approved by the Animal Care and Use Committee of the University of Colorado. Biochemical analysis Biochemical analysis for ALT, AST, urea nitrogen, creatinine, total cholesterol, low-density lipoprotein cholesterol, high-density lipoprotein cholesterol, triglyceride, glucose, HbA1c and uric acid was done with an automated chemistry analyser (VetACE Clinical Chemistry System, Alfa Wassermann Diagnostic Technologies). The serum level of leptin and insulin was determined using a mouse leptin ELISA kit and Ultra Sensitive Mouse Insulin ELISA Kit (Crystal Chem), respectively. Liver fructose, sorbitol and β-hydroxybutyrate concentration was measured with EnzyChrom fructose assay kit (BioAssay Systems) and β-hydroxybutyrate and sorbitol assay kits (Biovision), respectively. Briefly, the sorbitol determination assay (Biovision) is based on the conversion of sorbitol to fructose with the generation of NADH (colour) through a recombinant SDH. Therefore, to avoid the effects from endogenous hepatic SDH, liver lysates are protein cleared through a 10-kDa spin column (Biovision) before analysing sorbitol levels with the kit. In contrast, the fructose assay kit is based in its metabolism by fructose dehydrogenase, an enzyme found only in plants but not mammals. For hepatic triglyceride determination, fat was solubilized by homogenization in 1 ml solution containing 5% nonidet P40 (NP‐40) in water; slowly, samples were exposed to 80–100 °C in a water bath for 2–5 min until theNP‐40 became cloudy, then were cooled down to room temperature. Samples were then centrifuged for 2 min to remove any insoluble material. Triglyceride determination with the VetAce autoanalyser consisted in their initial breakdown into fatty acids and glycerol. Glycerol is then oxidized to generate a product, which reacts with the probe to generate colour at 570 nm. Histopathology Paraffin-embedded sections were stained with either H&E or Mallory trichrome. Histological examination was performed using the procedures described by Brunt et al. [39] as modified by Kleiner et al., [40] and was expanded for use in rodents by Orlicky et al. [41] Briefly, for H&E staining, sections were deparaffined and passed dehydrated with xylenes and ethanol. Slides were thoroughly washed and dipped in haematoxylin, washed again with water and ethanol 95%, and incubated with eosin for 30 min. After incubation, sections were re-incubated with ethanol and xylenes, and were covered with mounting medium. For Mallory trichrome, slides were hydrated with xylenes and ethanol, and were stained with 1% fuchsin acid solution for 2 min. After incubation, slides were washed and stained with 1% phosphomolybdic acid solution, washed again and dipped into solution containing 2% Orange G, 0.5% methyl blue and 2% oxalic acid for 15 min. Slides were then washed thoroughly, dehydrated with ethanol/xylenes and were mounted. Images were captured on an Olympus BX51 microscope equipped with a four megapixel Macrofire digital camera (Optronics, Goleta, CA) using the PictureFrame Application 2.3 (Optronics). Composite images were assembled with the use of Adobe Photoshop. All images in each composite were handled identically. For oil red O staining, 0.3% Oil Red O solution (Sigma-Aldrich) was freshly prepared by mixing 0.5% Oil Red O solution dissolved in isopropanol and distilled water at a ratio of 3:2, and then filtered. Liver sections (4 μm thick) were cut with a cryostat, fixed in 10% formalin and washed with running water. Sections were rinsed with 60% isopropanol, stained with Oil Red O staining solution for 15 min and then rinsed with 60% isopropanol. Finally, sections were counterstained with haematoxylin and then examined under a light microscope. Immunostaining for AR and KHK was performed from deparaffinized sections. The sections were immunostained with the specific primary antibodies described in the text, followed by the appropriate secondary antibody labelled with either Alexa 488 or Alexa 594 (Molecular Probes, Eugene, OR) and nuclei were stained with DAPI (Sigma Chemical Company, St Louis, MO). Image analysis and CLD quantitation Immunofluorescence images were captured at room temperature on a Nikon Diaphot fluorescence microscope equipped with a Cooke SensiCam CCD camera (Tonawand, NY), using Slidebook software (Intelligent Imaging Innovations Inc., Denver, CO) as previously described [20] . Fluorescence images were digitally deconvolved using the No Neighbors algorithm (Slidebook) and converted to TIFF files. All images were processed and assembled into montages in Photoshop (Adobe Systems Inc., Mountain View, CA). Images shown in any one montage have been taken and processed similarly to allow visual comparisons of relative protein levels in cells expressing the same protein(s). Western blotting Protein lysates were prepared from mouse tissue employing mitogen-activated protein kinase lysis buffer as previously described [42] . Briefly, tissues (~50 mg) were homogenized in 500 μl of buffer containing 0.5% triton X-100, 2 mM MgCl 2 , 1 mM EGTA and 1 mM dithiothreitol supplemented with protease and phosphatase inhibitors (Roche); samples were then incubated on ice for 30 min with occasional vortex and spinned at 13,000 r.p.m. for 15 min at 4 o C. Supernatant was collected and content determined by the BCA protein assay (Pierce). Fifty micrograms of total protein was loaded per lane for SDS–PAGE (10% w/v) analysis and then transferred to polyvinylidene difluoride membranes. Membranes were incubated with primary antibodies (all of them at a 1:1,000 dilution; AR, custom-made raised in rabbit; SDH Proteintech 15881-1-AP; KHK, Sigma HPA007040; ACL, Cell Signaling 4332S; FAS, Cell Signaling 3180S) and were visualized using a horseradish peroxidase secondary antibody(1:2,000) and the HRP Immunstar detection kit (Bio-Rad, Hercules, CA). Chemiluminescence was recorded with an Image Station 440CF and results were analysed with the 1D Image Software (Kodak Digital Science, Rochester, NY). Cultured cells Human-derived hepatocyte cell line HepG2 cells were grown in 80% confluency in RPMI-1640 medium (Invitrogen) supplemented with 10% FCS and antibiotics. Once cells reached the confluency, they were exposed to glucose (20 mM) for 3 days, with fresh changes of medium twice daily in the presence or absence of sorbinil (10 μM, kindly provided by Pfizer Central Research, New York, NY). After 72 h, cells were lysed with 5% NP40 and exposed to 80–100 °C in a water bath for 2–5 min until the NP‐40 became cloudy, then were cooled down to room temperature. Samples were then centrifuged for 2 min to remove any insoluble material and triglyceride concentration determined with the VetAce autoanalyser. Statistical analysis All data are presented as the mean±s.e.m. Independent replicates for each data point ( n ) are identified in figure legends. Data graphics and statistical analysis were performed using Prism 5 (GraphPad). Data without indications were analysed by one-way analysis of variance, Tukey’s post hoc test. P <0.05 was regarded as statistically significant. How to cite this article: Lanaspa, M. A. et al. Endogenous fructose production and metabolism in the liver contributes to the development of metabolic syndrome. Nat. Commun. 4:2434 doi: 10.1038/ncomms3434 (2013).